Kctd10 regulates heart morphogenesis by repressing the transcriptional activity of Tbx5a in zebrafish The T-box transcription factor Tbx5 (Tbx5a in zebrafish) plays a crucial role in the formation of cardiac chambers in a dose-dependent manner. Its deregulation leads to congenital heart disease. However, little is known regarding its regulation. Here we isolate a zebrafish mutant with heart malformations, called 34c . The affected gene is identified as kctd10 , a member of the potassium channel tetramerization domain (KCTD)-containing family. In the mutant, the expressions of the atrioventricular canal marker genes, such as tbx2b , hyaluronan synthase 2 ( has2 ), notch1b and bmp4 , are changed. The knockdown of tbx5 rescues the ectopic expression of has2 , and knockdown of either tbx5a or has2 alleviates the heart defects. We show that Kctd10 directly binds to Tbx5 to repress its transcriptional activity. Our results reveal a new essential factor for cardiac development and suggest that KCTD10 could be considered as a new causative gene of congenital heart disease. During the development of the vertebrate embryo, the heart is the earliest organ to form and to function. The primitive heart is a simple tube containing only two layers: an outer myocardium and an inner endocardium. Cardiac jelly is localized between the two layers and occupies the majority of the wall of the heart tube [1] . Subsequently, the tube undergoes a series of complicated morphogenetic processes called heart looping to form the final multi-chambered heart [2] . The formation of the atrioventricular canal (AVC) is one of the most important steps. The AVC separates the linear heart tube into the initial atrial and ventricular chambers and the myocardial cells at the AVC proliferate slowly and retain a slow conduction velocity, which is critical for the establishment of synchronized beating in the embryonic heart [3] . In the last 20 years, several signalling pathways that control cardiac development have been identified in vertebrates, ranging from zebrafish to humans. All these signalling pathways guide cardiogenesis through a series of transcription factors, such as the GATA family, NK2 transcription factor-related 5 (Nkx2-5), the basic helix-loop-helix transcription factors dHand and MesP1, Kruppel-like factor, the T-box (Tbx) transcription factors and FoxN4 (refs 4 , 5 , 6 , 7 , 8 ). The critical roles of the T-box transcription factors are initially revealed by analysing the phenotypes of human congenital heart malformations. For example, TBX1 haploinsufficiency causes DiGeorge syndrome and TBX5 haploinsufficiency results in Holt-Oram syndrome [9] , [10] . Targeted mutagenesis or knockdown of the genes encoding the T-box transcription factors demonstrates that Tbx1, Tbx2, Tbx3, Tbx5 (Tbx5a in zebrafish), Tbx18 and Tbx20 play essential roles during cardiac development in the mice or zebrafish [11] , [12] , [13] , [14] , [15] , [16] , [17] , [18] , [19] . Tbx5 plays a crucial role in the formation of the cardiac chambers and the AVC. This protein synergistically acts with Tbx20, BMP4, GATA4, Nkx2-5 and other factors to regulate the expression of many chamber-specific genes [8] , [14] , [20] . It also restricts the expression of Tbx2 ( tbx2b in zebrafish) and has2 (hyaluronan synthase 2) at the AVC to facilitate the formation of the endocardial cushion and valve [21] . Deregulation of has2 abrogates the normal cardiac morphogenesis [22] , [23] . Abnormal cardiac morphogenesis is closely correlated with the dose of Tbx5 (refs 24 , 25 ). Holt-Oram syndrome occurs in heterozygous individuals, whereas homozygous-null mutations in Tbx5 exhibit very severe heart malformations. Tbx5 duplication or overexpression results in phenotypes similar to the Holt-Oram syndrome [26] . These data indicate that the expression level and/or the activity of Tbx5 are precisely controlled during heart development. However, the mechanism of the regulation of Tbx5 is poorly understood. In this study, we isolate a zebrafish mutant with heart malformations, called 34c . On the basis of positional cloning, the affected gene is identified as kctd10 , a member of the potassium channel tetramerization domain (KCTD) containing family. KCTD proteins comprise a large family containing at least 22 members in human, but only several members have been studied. Because KCTD genes have not been targeted in any model organisms, their precise roles in development are unknown. Here we demonstrate that Kctd10 protein controls cardiac development by directly binding to Tbx5 to repress its transcriptional activity. Therefore, Kctd10 plays an essential role in cardiac development, which could be considered as a new candidate for the genetic screening of congenital heart diseases in the future. kctd10 deficiency leads to heart defects in the mutant 34c We identified a spontaneous recessive mutation called 34c that disrupted cardiac function in zebrafish. This mutant exhibited AVC malformations and heart looping failure. The mutants were indistinguishable from their siblings until ~36 hpf (hours post fertilization), when heart looping starts [8] , [27] . Thereafter, approximately one-fourth of the embryos displayed heart looping defects, then weakened heart contractility, weakening circulation, an accumulation of blood cells in the venous sinus, and pericardial oedema at 48 hpf ( Fig. 1a,b ). The hearts of their wild-type siblings beat normally at 48 hpf ( Supplementary Movie 1 ). In contrast, the atrium of the 34c mutant appeared to have very weak contractility and a slower heart rate. However, global contraction still occurred and no fibrillation or arrhythmia was observed. The ventricle became completely still at 48~52 hpf ( Supplementary Movie 2 ). 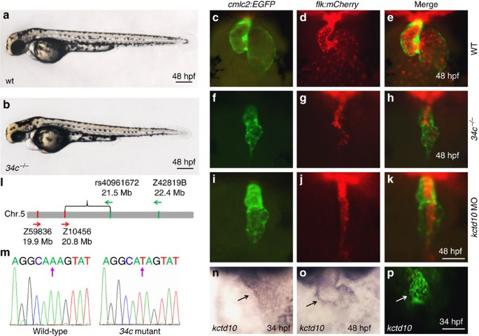Figure 1:Kctd10is responsible for the heart defect of the zebrafish mutant34c. (a,b) Bright-field micrographs of wild-type (wt) and34cmutant embryos at 48 hpf. The mutant exhibits certain pericardial oedema. Scale bars=0.25 mm. (c–k) Fluorescence micrographs of the hearts of wild-type (c–e),34cmutant (f–h) and embryos injected with 4 ng MO against the translation ofkctd10(i–k) at 48 hpf under the background ofTg(cmlc2:EGFP)/Tg(flk:mCherry)transgenic fish. Both the myocardium (green) and the endocardium (red) are substantially smaller in the mutant and the morphant, and no cavity is visible inside the heart lumen. Scale bar=0.1 mm. (l) A genetic map of the34cmutant placed the affected gene between markersZ10456(Chr5: 20.84 Mb) andrs40961672(Chr5: 21.47 Mb) (Ensembl Zv9). (m) Sequencing result ofkctd10cDNA revealed an A-to-T transversion at position 120 of exon 2. (n,o)In situhybridization ofkctd10in wild-type embryos.Kctd10was expressed in the heart (arrow) at 34 and 48 hpf. (p) Kctd10 protein detected by immunofluorescence. The heart tube is indicated by arrow. (n–p) Scale bar=0.1 mm. (c–k,n–p) Ventral views with the anterior at the top. Figure 1: Kctd10 is responsible for the heart defect of the zebrafish mutant 34c . ( a , b ) Bright-field micrographs of wild-type (wt) and 34c mutant embryos at 48 hpf. The mutant exhibits certain pericardial oedema. Scale bars=0.25 mm. ( c – k ) Fluorescence micrographs of the hearts of wild-type ( c – e ), 34c mutant ( f – h ) and embryos injected with 4 ng MO against the translation of kctd10 ( i – k ) at 48 hpf under the background of Tg(cmlc2:EGFP)/Tg(flk:mCherry) transgenic fish. Both the myocardium (green) and the endocardium (red) are substantially smaller in the mutant and the morphant, and no cavity is visible inside the heart lumen. Scale bar=0.1 mm. ( l ) A genetic map of the 34c mutant placed the affected gene between markers Z10456 (Chr5: 20.84 Mb) and rs40961672 (Chr5: 21.47 Mb) (Ensembl Zv9). ( m ) Sequencing result of kctd10 cDNA revealed an A-to-T transversion at position 120 of exon 2. ( n , o ) In situ hybridization of kctd10 in wild-type embryos. Kctd10 was expressed in the heart (arrow) at 34 and 48 hpf. ( p ) Kctd10 protein detected by immunofluorescence. The heart tube is indicated by arrow. ( n – p ) Scale bar=0.1 mm. ( c – k , n – p ) Ventral views with the anterior at the top. Full size image In the mutant embryos at 36 hpf, no marked differences were observed when compared with wild-type, but the mutants had markedly smaller eyes and smaller heads at 48 hpf ( Fig. 1a,b ; supplementary Fig. 1a–d ). Moreover, the pectoral fins of the mutant larvae were smaller than their normal siblings ( Supplementary Fig. 1e–j ). To further investigate the cardiac malformations, we analysed the 34c mutant under the backgrounds of two transgenic fish lines: Tg ( cmlc2:EGFP ) that labels the myocardium, and Tg ( flk:mCherry ) that labels the endocardium. As visualized using these transgenic lines, both the myocardium and the endocardium of the chambers in the mutants were markedly shrunken and the heart failed to loop normally compared with the wild-type siblings ( Fig. 1c–h ). The endocardium was more severely reduced than the myocardium, with nearly no lumen present ( Fig. 1g,h ). The defect became increasingly severe over time. The oedema of the venous sinus appeared at 50 hpf and the mutant died at ~5 dpf (days post fertilization). However, the patterns of blood vessels in the mutants were indistinguishable from that in the wild-type siblings ( Supplementary Fig. 2 ). We performed positional cloning to identify the affected gene that caused the phenotype of 34c . Meiotic mapping of 34c identified a 0.63-Mb interval between rs40961672 (LG (linkage group) 5: 21 468 103 bp) and Z10456 (LG5: 20838789–20838997, bp) of chromosome 5 ( Fig. 1l ). The annotated Ensembl zebrafish genome assembly Zv9 suggested 10 candidate genes in this region. After sequencing the coding region of these candidate genes, a homozygous A-to-T substitution at position 120 of exon 2 of the gene kctd10 was identified in the 34c mutants ( Fig. 1m ). This change replaced Lysine (AAG) with a pre-mature stop codon (TAG) at amino-acid position 113. The tetramerization domain of Kctd10 is located within its N-terminus, and the truncation by the nonsense mutation eliminates part of this domain. When we in-crossed the kctd10 +/− fish, it always resulted in 25% of the embryos displaying the mutant phenotype. No obvious dominant-negative activity was observed. To confirm that the deficiency of kctd10 was responsible for the phenotype of 34c −/− , we injected kctd10 mRNA into one-cell stage zebrafish embryos derived from the in-cross of 34c +/− and found that the ratio of the mutant embryos was significantly less than 25% ( P <0.01 by the χ 2 test.) ( Supplementary Fig. 3 ). The wild-type embryos injected with kctd10 mRNA were indistinguishable from the wild-type embryos injected with phosphate-buffered saline (PBS). The injection of a morpholino (MO) against the translation of kctd10 into wild-type embryos resulted in a phenotype that was indistinguishable from the 34c mutant ( Fig. 1h,i , Supplementary Movie 3 ). More importantly, we targeted kctd10 in zebrafish by TALEN (transcription activator-like effector nucleases) and obtained F 1 fish with an 8 bp-deletion in exon3 of kctd10 at one allele ( kctd10 +/TALEN ). About one-fourth of the offspring derived from the in-cross between kctd10 +/TALEN showed the same phenotype as 34c mutant. Complementation testing revealed that about one-fourth of the larvae (10/41 and 13/58 in two independent assays) from the cross between kctd10 +/TALEN and 34c +/− showed phenotypes very similar to 34c mutants ( Supplementary Fig. 4 ). These data demonstrate that the nonsense mutation of kctd10 is responsible for the phenotype of the 34c mutant. Zebrafish Kctd10 protein is composed of 313 amino-acid residues and shares 94% identity with its orthologues in humans and mice ( Supplementary Fig. 5 ). In situ hybridization revealed that kctd10 mRNA was present in embryos at the one-cell stage, and its expression was ubiquitous until 24 hpf ( Supplementary Fig. 6 ). At 34 hpf, kctd10 was detected in the heart tube, the brain and the hatching gland ( Fig. 1n ; Supplementary Fig. 6 ). At 48 hpf, its expression was maintained in both the atrium and ventricle ( Fig. 1o ). Kctd10 protein was also present in the heart tube at 34 hpf ( Fig. 1p ). Kctd10 is required for AVC formation We investigated the expression of several common cardiac markers by in situ hybridization in kctd10 mutants. At 18 hpf, when the myocardial precursors segregate into two populations adjacent to the midline, the expression of the heart tube marker cmlc2 (cardiac myosin light chain 2) did not differ between the mutant and the wild-type ( Supplementary Fig. 7a,b ). These data suggest that the specification of the cardiac mesoderm is not affected in the mutant. The expression of cmlc2 also showed no difference at 48 hpf ( Supplementary Fig. 7c,d ). The ventricular marker vmhc (ventricular myosin heavy chain) and the atrial marker amhc (atrial myosin heavy chain, also known as myh6 ) were used to visualize the two chambers, respectively. At 48 hpf, amhc was detected in the atria of both the wild-type and mutant larvae ( Supplementary Fig. 7e,f ). Vmhc was detected in the ventricles of both the wild-type and mutant embryos ( Supplementary Fig. 7g,h ). The cardiac mesoderm marker nkx2.5 was also examined and no difference was found between the kctd10 mutants and their wild-type siblings ( Supplementary Fig. 7i,j ). In contrast to the early genes necessary for cardiogenesis, the expression of the AV boundary marker genes, such as bmp4 , notch1b , tbx2b and has2 , was dramatically affected in the kctd10 mutants. At 34 hpf, the expression patterns of bmp4 , notch1b and tbx2b showed no difference between the mutants and the control embryos ( Fig. 2a,b,e,f,i,j ). In the heart of wild-type embryos at 48 hpf, bmp4 , notch1b and tbx2b were expressed at the prospective AVC ( Fig. 2c,g,k ). However, bmp4 and tbx2b expanded throughout the myocardium ( Fig. 2d,l ), and notch1b expanded over the entire endocardium in the mutant ( Fig. 2h ). 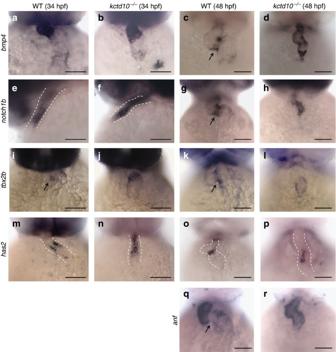Figure 2: The atrioventricular canal is malformed in thekctd10mutant. The expression ofbmp4,notch1b,tbx2b, has2andanfin wild-type andkctd10mutant embryos at 34 and/or 48 hpf was shown byin situhybridization. The expression patterns ofbmp4, notch1bandtbx2bdid not differ dramatically between the mutant and wild-type embryos at 34 hpf (a,b,e,f,i,j), but showed significant difference at 48 hpf (c,d,g,h,k,l).Has2were localized to a restricted region in wild-type embryos (m,o), while its expression expanded significantly in the mutant, especially at 34 hpf (n,p) The border of the heart is delineated with the dotted lines. The expression ofanfwas also upregulated and detected in the AVC in the mutant (q,r; the arrow inqindicates the AVC.) at 48 hpf. (a–d,g–r) Ventral views with the anterior at the top; (e,f) Lateral views with the anterior to the left. Scale bars=0.1 mm. Figure 2: The atrioventricular canal is malformed in the kctd10 mutant. The expression of bmp4 , notch1b , tbx2b, has2 and anf in wild-type and kctd10 mutant embryos at 34 and/or 48 hpf was shown by in situ hybridization. The expression patterns of bmp4, notch1b and tbx2b did not differ dramatically between the mutant and wild-type embryos at 34 hpf ( a , b , e , f , i , j ), but showed significant difference at 48 hpf ( c , d , g , h , k , l ). Has2 were localized to a restricted region in wild-type embryos ( m , o ), while its expression expanded significantly in the mutant, especially at 34 hpf ( n , p ) The border of the heart is delineated with the dotted lines. The expression of anf was also upregulated and detected in the AVC in the mutant ( q , r ; the arrow in q indicates the AVC.) at 48 hpf. ( a – d , g – r ) Ventral views with the anterior at the top; ( e , f ) Lateral views with the anterior to the left. Scale bars=0.1 mm. Full size image Has2 is essential for AVC formation [21] , [22] , [23] . Its expression was detected at the AVC region in the wild-type embryos ( Fig. 2m,o ); In the kctd10 mutant embryos at 48 hpf, expression of has2 expanded ( Fig. 2p ). More impressively, the ectopic expression of has2 in the mutant embryos at 34 hpf was more remarkable than in the mutants at 48 hpf ( Fig. 2n ). As mentioned above, the mutant embryos before 36 hpf was indistinguishable from their siblings. These results indicate that the ectopic expression of has2 occurs before the emergence of the phenotype. In the mutant, the myocardial chamber marker anf , also known as nppa (natriuretic peptide type A), was also upregulated and detected throughout the entire heart, including the AVC ( Fig. 2q,r ). The altered expression of these AVC marker genes indicates that the AVC in the kctd10 mutant is malformed. The mutations of the genes encoding the ion channel proteins usually result in heart malformations. To identify whether Kctd10 protein acts as a potassium channel, the K + flux around the surface of the heart was measured by the Scanning Ion-selective Electrode Technique (SIET). The K + showed net influx at the heart surface. No significant difference was detected between the kctd10 mutants and their normal siblings ( Supplementary Fig. 8 ). Moreover, we have treated the kctd10 mutant embryos with the drugs that could alter the heart contractility and/or heart rate, such as adrenaline, digilanid and atropine. Adrenaline increases the heart rate and elevates blood pressure. Digilanid increases myocardial contractility and blood pressure while reducing heart rate. Atropine is a muscarinic acetylcholinergic antagonist that increases firing of the sinoatrial node and conduction through the atrioventricular node of the heart. Both adrenaline and atropine increased the heart rates in both the wild-type and the mutant zebrafish embryos, while digilanid reduced the heart rate, as expected. However, none of the drugs were able to relieve the cardiac morphology of the mutant ( Supplementary Fig. 9 ). These data demonstrate that the heart defects of kctd10 mutant are unlikely due to the physical forces. Knockdown of has2 alleviates the phenotype in the mutant Has2 protein is the synthetase of hyaluronic acid, an extracellular glycosaminoglycan that is the major component of the cardiac jelly. Ectopic expression of Has2 is reported to impair cardiac looping, results in lumen narrowing and increases the space between the endocardium and myocardium in the heart chambers [22] . This phenotype was also observed in the histological sections of kctd10 mutants at 48 hpf ( Fig. 3a,f ). We stained hyaluronic acid by biotinylated hyaluronan-binding protein. The layer of hyaluronic acid in the cardiac jelly of the mutant was much thicker than that of the wild-type ( Fig. 3b–j ). 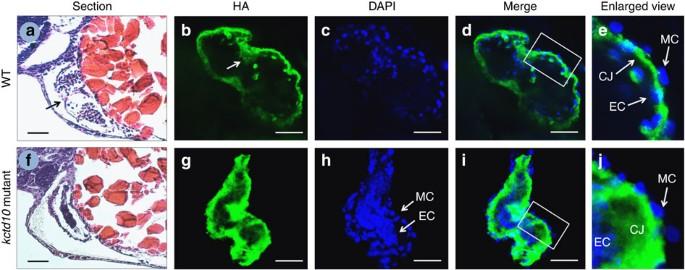Figure 3: The cardiac jelly in the34cmutant becomes thicker. (a,f), Histological sections of hearts from wild-type and mutant embryos at 48 hpf, staining with H&E. The endocardium of the mutant was extremely shrunken and the space between the myocardium and endocardium was much wider than that of the wild-type. The AVC (a, arrow) disappeared in the mutant (f). (b–j) Hyaluronic acid staining (green) and nucleus staining (blue) of the hearts of wild-type (b–e) andkctd10mutant (g–j) embryos at 48 hpf. The arrow inbindicates the endocardial cushions at AVC, where more HA is localized. (e,j) enlarged views of the atrium wall (boxed ind,i). CJ, cardiac jelly; EC, endocardial cells nuclei; MC, myocardial cells nuclei. Scale bars=0.05 mm. Figure 3: The cardiac jelly in the 34c mutant becomes thicker. ( a , f ), Histological sections of hearts from wild-type and mutant embryos at 48 hpf, staining with H&E. The endocardium of the mutant was extremely shrunken and the space between the myocardium and endocardium was much wider than that of the wild-type. The AVC ( a , arrow) disappeared in the mutant ( f ). ( b – j ) Hyaluronic acid staining (green) and nucleus staining (blue) of the hearts of wild-type ( b – e ) and kctd10 mutant ( g – j ) embryos at 48 hpf. The arrow in b indicates the endocardial cushions at AVC, where more HA is localized. ( e , j ) enlarged views of the atrium wall (boxed in d , i ). CJ, cardiac jelly; EC, endocardial cells nuclei; MC, myocardial cells nuclei. Scale bars=0.05 mm. Full size image Cardiac jelly is essential for cardiac development, including the AVC formation and heart looping [28] , [29] , [30] . To clarify whether the ectopic expression of has2 was the cause of the heart defect in the kctd10 mutant, the MO against has2 was injected into the embryos derived from the in-cross of Tg(cmlc2:EGFP) 34c+/− fish. At 48 hpf, only 10% (6/59) of the embryos injected with 6 ng per embryo of has2 MO had the same phenotype as the kctd10 mutant ( Supplementary Table 1 ). The hearts of the majority of the embryos were not shrunken, but the AVC became wider than that of the wild-type as described before [23] ( Fig. 4a,b ). The heart of these morphants exhibited a sequential, coordinated beating of the atrium and ventricle ( Supplementary Movie 4 , genotyped as wild-type). Functional circulation was also observed. Eight out of 59 embryos seemed to have normal cardiac morphogenesis and circulation. These eight embryos were genotyped and five of them were kctd10 mutants ( Fig. 4e ; Supplementary Movie 5 ). 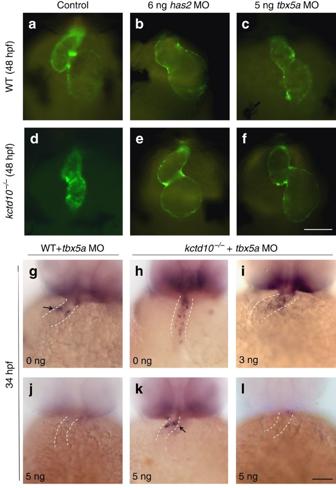Figure 4: The knockdown ofhas2ortbx5aalleviates the heart defect inkctd10mutants. (a–f) The MO againsthas2ortbx5awas injected into the embryos derived from the in-cross ofTg(cmlc2:EGFP)+/34cfish. The heart of thekctd10mutant (d) was markedly smaller than the wild-type embryos (a) at 48 hpf. The AVC of wt embryos injected withhas2MO became wider (b), and the heart of wt embryos injected withtbx5aMO is slightly shrunken (c). (e,f) Some injected mutants have nearly normal cardiac morphogenesis. (g–l)In situhybridization ofhas2in the mutants injected withtbx5aMO.Has2was expressed in the very restricted region of the endocardium in wild-type embryos (g, arrow), whereas it expanded throughout the endocardium of the heart tube in thekctd10mutants (h). When treated with 3 ng oftbx5aMO, the ectopic expression ofhas2decreased moderately in some mutants (i); in case of injection with 5 ng oftbx5aMO,has2was undetectable in wild-type embryo (j), but restricted at the AVC in 5/16 mutants (k, arrow); in 3/16 mutants,has2disappeared (l). All the embryos used here were genotyped. Ventral views with the anterior at the top. (a–f) Scale bar=0.1 mm; (g–l) Scale bar=0.1 mm. Figure 4: The knockdown of has2 or tbx5a alleviates the heart defect in kctd10 mutants. ( a – f ) The MO against has2 or tbx5a was injected into the embryos derived from the in-cross of Tg(cmlc2:EGFP) +/34c fish. The heart of the kctd10 mutant ( d ) was markedly smaller than the wild-type embryos ( a ) at 48 hpf. The AVC of wt embryos injected with has2 MO became wider ( b ), and the heart of wt embryos injected with tbx5a MO is slightly shrunken ( c ). ( e , f ) Some injected mutants have nearly normal cardiac morphogenesis. ( g – l ) In situ hybridization of has2 in the mutants injected with tbx5a MO. Has2 was expressed in the very restricted region of the endocardium in wild-type embryos ( g , arrow), whereas it expanded throughout the endocardium of the heart tube in the kctd10 mutants ( h ). When treated with 3 ng of tbx5a MO, the ectopic expression of has2 decreased moderately in some mutants ( i ); in case of injection with 5 ng of tbx5a MO, has2 was undetectable in wild-type embryo ( j ), but restricted at the AVC in 5/16 mutants ( k , arrow); in 3/16 mutants, has2 disappeared ( l ). All the embryos used here were genotyped. Ventral views with the anterior at the top. ( a – f ) Scale bar=0.1 mm; ( g – l ) Scale bar=0.1 mm. Full size image We also coinjected has2 MO and kctd10 MO into the wild-type embryos. Compared with the embryos injected with only kctd10 MO, neither the myocardium nor the endocardium of 90% (50/56) embryos injected with both MOs showed a substantial decrease in size. More importantly, the heart looping in >20% (12/56) of the double morphants was recovered completely ( Supplementary Fig. 10 ), whereas in 60% (38/56) double morphants, the heart looping was partially recovered and showed more mature hearts than in the kctd10 morphants. The heart of the majority of the double morphants exhibited a sequential, coordinated beating of the atrium and ventricle. In summary, repressing the expression of has2 in kctd10 mutants/morphants resulted in the recovery of the heart defects. Considering that the ectopic expression of has2 occurs before the emergence of the phenotype, these data demonstrate that the ectopic expression of has2 is the major cause of heart malformations in the kctd10 mutants. Knockdown of tbx5a alleviates heart defects in kctd10 mutant We wanted to determine what causes the ectopic expression of has2 . We noticed that the phenotype of kctd10 mutant, including the shrunken heart, the slower heart rate and the smaller pectoral fin, was similar to the zebrafish mutant heartstrings [31] . Thus, the expression of tbx5a was examined by in situ hybridization. Unexpectedly, the expression pattern of tbx5a in the mutants revealed no marked differences from the wild-type embryos ( Supplementary Fig. 11 ). Also unexpectedly, injection of tbx5a mRNA was not able to rescue the phenotype of the mutants. Considering that Tbx5 overexpression resulted in a similar phenotype to Tbx5 deficiency [26] , we injected the MO against tbx5a into the embryos derived from the in-cross of the Tg(cmlc2:EGFP) 34c+/− zebrafish strain. When we injected 3 ng of tbx5a MO, 13 out of 60 embryos exhibited the kctd10 mutant phenotype, but 6 out of the 13 embryos showed weakened circulation at 48 hpf. The expression of has2 in these mutants was also mildly decreased, indicating partial rescue ( Supplementary Tables 1,2 ; Supplementary Fig. 12c ). When 5 ng of tbx5a MO was injected into each embryo, the observed number of embryos with the mutant phenotype at 48 hpf was far less than expected (8/66) ( Supplementary Table 1 ). Nine injected embryos had normal cardiac morphogenesis. These embryos were genotyped and eight of them were kctd10 mutants ( Fig. 4f ; Supplementary Movie 6 ). The expression pattern of has2 was also rescued in the mutants with normal phenotype ( Supplementary Fig. 12e ). Functional circulation was observed in these embryos. The hearts of the majority of the embryos shrank slightly, but exhibited a sequential, coordinated beating ( Fig. 4c ; Supplementary Movie 7 , genotyped as wild-type). In the embryos with slightly shrunken hearts (12 of these embryos were genotyped and one was mutant), the expression of has2 was not detected ( Supplementary Fig. 12d,f ). We also injected 6 ng of tbx5a MO into the embryos of kctd10 mutants, and obtained the similar results ( Supplementary Table 1 ). As mentioned above, the ectopic expression of has2 is the major cause of heart malformations in the kctd10 mutants. Now that knock down of tbx5a was able to rescue the heart malformations in kctd10 mutants, tbx5a MO should also rescue the ectopic expression of has2 in the mutants at 34 hpf. Thus, we examined the expression of has2 in kctd10 mutants injected with tbx5a MO at 34 hpf. With the injection of 3 ng of tbx5a MO, has2 was decreased in 6 out of 15 mutants, indicating partial rescue ( Fig. 4i ; Supplementary Table 2 ). In the rest nine mutants, the expression of has2 was similar to that in the mutant injected with PBS. When injected with 5 ng of tbx5a MO, the expression of has2 was restricted at the AV junction in 5 out of 16 mutants at 34 hpf; in 3 out of the 16 mutants, has2 disappeared ( Fig. 4k,l ; Supplementary Table 2 ). Thus, knockdown of tbx5a could rescue both the heart malformations and the ectopic expression of has2 in kctd10 mutants. The MO against tbx5a was also coinjected into wild-type embryos with the MO against kctd10 . When 3 ng of tbx5a MO was injected into the embryos together with the kctd10 MO, the expression of has2 was recovered to normal in 8 out of 30 embryos. The ectopic expression of has2 was moderately reduced in the other 22 embryos, indicating partial rescue ( Supplementary Fig. 12h,i ; Supplementary Table 2 ). When the dosage of 5 ng per embryo was used, the ectopic expression of has2 was eliminated in 10 out of 24 samples, and has2 expression disappeared in 14 out of 24 embryos ( Supplementary Fig. 12k,l ; Supplementary Table 2 ). These data suggest that Tbx5a is hyperactivated in the kctd10 mutants/morphants, although the expression of tbx5a does not alter much. It indicates that Kctd10 protein may play a role in repressing the transcriptional activity of Tbx5a. Considering that the dosage of Tbx5/5a is critical for cardiac morphogenesis and we could not control the dosage of tbx5a MO exactly, the knockdown of tbx5a did not rescue the cardiac malformations in all mutants/morphants. Kctd10 directly binds to Tbx5/5a to repress its activity To confirm that Kctd10 protein moderated the transcriptional activity of Tbx5, the reporter construct of G5E1b-luciferase and the expression vector Gal4-Tbx5(266–518) were used for reporter assay. G5E1b-luciferase contains five Gal4-binding elememts [32] and Gal4-Tbx5(266-518) contains the coding sequences of the Gal4 DNA-binding domain fused to Tbx5 transactivating domain in-frame [33] . The transactivating domain of Tbx5 dramatically stimulated the expression of the Luciferase gene (>600-fold). This strong activation was significantly suppressed by the expression of Kctd10 in a dose-dependent manner ( Fig. 5a ). In contrast, Kctd10 had no effect on the activity of G5E1b-luciferase induced by Gal4-VP16 ( Fig. 5a ). 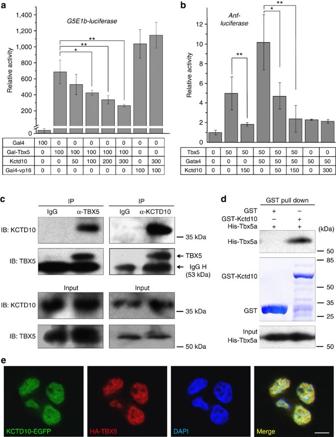Figure 5: Kctd10 directly binds to Tbx5/5a to moderate its transcriptional activity. (a,b) Luciferase reporter assays of theG5E1band the 0.7-kbAnfpromoter fragment. Numbers indicate the quantity (nanograms) of each corresponding plasmid. At least three independent experiments were performed for each assay, and each in quadruplicate (mean±s.e.m.;n=4). Asterisks represent the statistical significance as determined using a Student’st-test (*P<0.05; **P<0.01). (c) Co-IP of endogenous TBX5 and endogenous KCTD10 in HeLa cells. (d) Pull-down assay of His-tagged Tbx5a by GST fusion Kctd10 protein bound to GSH-agarose beads and subsequent detection by western with anti-His antibody. The expression of GST and GST fusion protein was stained by Coomassie brilliant blue. (e) Immunofluorescent detection of HA-Tbx5a and Kctd10-GFP in 293T cells. Nuclei are counterstained by DAPI. Scale bar=10 μm. Figure 5: Kctd10 directly binds to Tbx5/5a to moderate its transcriptional activity. ( a , b ) Luciferase reporter assays of the G5E1b and the 0.7-kb Anf promoter fragment. Numbers indicate the quantity (nanograms) of each corresponding plasmid. At least three independent experiments were performed for each assay, and each in quadruplicate (mean±s.e.m. ; n =4). Asterisks represent the statistical significance as determined using a Student’s t -test (* P <0.05; ** P <0.01). ( c ) Co-IP of endogenous TBX5 and endogenous KCTD10 in HeLa cells. ( d ) Pull-down assay of His-tagged Tbx5a by GST fusion Kctd10 protein bound to GSH-agarose beads and subsequent detection by western with anti-His antibody. The expression of GST and GST fusion protein was stained by Coomassie brilliant blue. ( e ) Immunofluorescent detection of HA-Tbx5a and Kctd10-GFP in 293T cells. Nuclei are counterstained by DAPI. Scale bar=10 μm. Full size image We also examined whether Kctd10 could regulate the expression of a Tbx5 target gene. Luciferase reporter assays were performed with the constructs of Anf(−0.7k)-Luc, where Luciferase is driven by the regulatory region of mouse Anf [2] , [33] . The results showed that the activation of Anf(−0.7k)-Luc mediated by Tbx5 was markedly suppressed by Kctd10 in a dose-dependent manner ( Fig. 5b ). Kctd10 had no effect on the transactivation of Anf mediated by Gata4 alone ( Fig. 5b ). Co-transfection of Kctd10 also repressed the Tbx5-Gata4-mediated activation of the Tbx2(−5.6/+0.316)-Luc in a dose-dependent manner, whereas Kctd10 had no significant effect on either Bmp/Smad-mediated transactivation or TBX20-mediated suppression of Tbx2 ( Supplementary Fig. 13a–c ). The expressions of Tbx5a target genes, including amhc ( myh6 ), tbx2b and anf , were also examined by real-time reverse transcriptase–PCR or deep sequencing. The results showed that all these genes were upregulated in the kctd10 mutant ( Supplementary Fig. 13d,e ; Supplementary Data 1 ). Thus, Kctd10 suppresses Tbx5a activity in vivo . How does Kctd10 protein moderate the transcriptional activity of Tbx5? We performed co-immunoprecipitation (Co-IP) experiments to investigate their association. The precipitation of Flag-Kctd10 protein was able to pull down Tbx5a from the cell lysate, and the precipitation of HA-Tbx5a was able to pull down Kctd10 ( Supplementary Figs. 13f and 15 ). HA-Tbx5a could also pull down endogenous KCTD10 ( Supplementary Figs. 13g and 15 ). The association between KCTD10 and TBX5 proteins was also confirmed in vivo . Immunoprecipitation of endogenous TBX5 with a polyclonal antibody against this protein specifically retrieved endogenous KCTD10 in HeLa cells, but not with the control immunoglobulin G of the rabbit. Consistently, anti-KCTD10 antibody was able to pull down TBX5 in the reciprocal co-IP assays ( Fig. 5c ; Supplementary Fig. 14 ). Thus, KCTD10 binding to TBX5 occurred in a cellular context. In vitro pull-down assays with glutathione S-transferase (GST)-Kctd10 fusion proteins was performed. These results show that Kctd10 protein directly binds to Tbx5a ( Fig. 5d ; Supplementary Fig. 14 ). To determine the cellular localization of Kctd10 protein, the fusion constructs of pEGFP-N1-KCTD10 and pRK-TBX5-HA were co-transfected into cells. The proteins were detected by green fluorescent protein (GFP)/immunofluorescence. The results showed the nuclear distribution of both KCTD10 and TBX5. KCTD10 protein colocalized with TBX5 in the nuclei ( Fig. 5e ). These results reveal that Kctd10 protein directly binds to Tbx5/5a to moderate its transcriptional activity in the nucleus. KCTD proteins comprise a large family and show high conservation across species. Few members of this family have been studied, aside from the following examples: KCTD5 mediates protein degradation in the proteasome [34] ; KCTD 8, 12 and 16 regulate the function of GABA B [35] ; KCTD15 suppresses canonical Wnt signalling through an unidentified mechanism [36] ; and KCTD10 interacts with proliferating cell nuclear antigen and DNA polymerase δ to regulate cell proliferation [37] , [38] . Recently, KCTD13 has been shown to relate to the copy number variant of 16p11.2 (ref. 39) [39] . Therefore, the functions of the KCTD proteins are quite diverse. However, KCTD genes have not been targeted in any model animals, and thus their roles in development are unknown. Here we demonstrate that Kctd10 plays a key role in cardiac morphogenesis via repressing the transcriptional activity of Tbx5. Tbx5 is a dose-sensitive transcription factor, so it needs to be tightly regulated. Very little is known about its regulation. JAK-STAT3 signalling is important for the expression of Tbx5, whereas PDZ and LIM domain protein 7 (Pdlim7) inactivates Tbx5 by tethering it in the cytoplasm [40] . Tbx20 also antagonizes Tbx5 function by repressing its expression [32] . Our data reveal a new mechanism of the regulation of Tbx5. Kctd10 physically binds to Tbx5 to modify the activity of the transactivating domain rather than control Tbx5 expression. Since Kctd10 and Tbx5 are colocalized in the nucleus, Kctd10 might be involved in the protein complex formed by Tbx5 and other factors, such as Tbx20, Nkx2.5 and Gata4. This regulation of Tbx5 is critical to restrict the expression of has2 , one of the critical genes for the formation of AVC, in the specific region of the heart tube. The ectopic expression of has2 causes heart malfornations [8] , [22] , that are very similar to the phenotype of kctd10 mutant. We confirmed that the heart defect in kctd10 mutant is due to the ectopic expression of has2 . On the basis of our findings and others’ previous work, we present a model to delineate the role of Kctd10 in heart morphogenesis ( Fig. 6 ). In the developing heart of the wild-type zebrafish embryo, the transcriptional activity of Tbx5 is moderated by Kctd10 to maintain its activity at a proper level. Tbx5 synergistically acts with other factors, such as BMP4, Nkx2.5, Gata4 and Tbx20, to restrict the expression of has2 at the AV boundary of the heart tube. Has2 catalyses the synthesis of hyaluronic acid, the major component of cardiac jelly, thus the cardiac jelly swells at the AVC. Has2 also plays a pivotal role in the epithelium-to-mesenchyme transformation of the endocardium at the AV boundary, which gives rise to the endocardial cushions and valves [22] , [23] , [27] . In the forming heart of the kctd10 mutant, Tbx5 is hyperactive due to the absence of functional Kctd10. As a result, has2 is no longer restricted to the AV boundary, but expands throughout the heart tube. The ectopic expression of has2 results in excess hyaluronic acid between the myocardium and endocardium, causing the cardiac jelly to swell throughout the entire heart tube. The excessive cardiac jelly affects the cross-talk between the myocardium and endocardium to cause the heart malformations [23] , [27] , [41] . 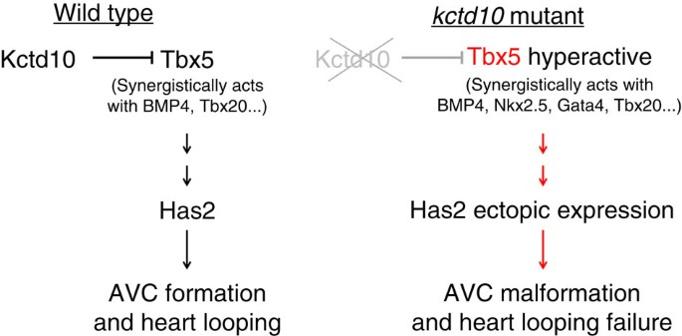Figure 6: A model of Kctd10 function in cardiogenesis. In wild-type zebrafish embryos, the transcriptional activity of Tbx5 is moderated by Kctd10, and Tbx5 synergistically acts with other factors to restricthas2at the prospective AVC region. When Kctd10 is deficient, Tbx5 is hyperactive to result in the ectopic expression ofhas2. Excess hyaluronic acid is deposited between myocardium and endocardium throughout the heart tube to lead to the malformations of AVC and heart looping failure. Figure 6: A model of Kctd10 function in cardiogenesis. In wild-type zebrafish embryos, the transcriptional activity of Tbx5 is moderated by Kctd10, and Tbx5 synergistically acts with other factors to restrict has2 at the prospective AVC region. When Kctd10 is deficient, Tbx5 is hyperactive to result in the ectopic expression of has2 . Excess hyaluronic acid is deposited between myocardium and endocardium throughout the heart tube to lead to the malformations of AVC and heart looping failure. Full size image In summary, we have isolated a zebrafish mutant strain with heart malformations and found that kctd10 is the affected gene. The Kctd10 protein plays a key role in restricting the expression of has2 to the AVC by directly binding to Tbx5 to moderate its transcriptional activity. Since Kctd10 and Tbx5 are colocalized in the nucleus, Kctd10 is likely to act as a co-repressor of Tbx5 epigenetically. Therefore, Kctd10 is an important factor for cardiac development, which may be considered as a new candidate for the genetic screening and identification of congenital heart diseases in the future. Zebrafish maintenance All the experimental procedures followed the rules of the Committee on Animal Care of Beijing, China (5 June 2008). All animal experiments were approved by Institutional Animal Care and Use Committee (IACUC) of Peking University. The reference from IACUC of Peking University is LSC-ZhangB-1. Zebrafish were raised and maintained at 28 °C in a circulating system that continuously filters, UV treats and aerates the circulating water. The in-tank breeding was used to obtain the embryos. The embryos were collected and raised in the incubator at 28 °C. The microinjection was performed at the one-cell stage. The larvae were anesthetized with 0.16 mg ml −1 Tricaine (MS-222, ethyl-3-aminobenzoate methanesulfonate salt, Sigma-Aldrich Inc.) before use [42] . Expression vectors and reporter plasmids The pAC-CMV-Tbx5 , Gal4-Tbx5-(266–518) , pAC-CMV-Tbx20 , pMT2-GATA4 , Gal4-VP16 expression plasmids and the G5E1b-luciferase reporter plasmids were kindly provided by Dr Katherine E. Yutzey [33] . The reporter plasmid of Tbx2(5.6/−0.316)-Luciferase was kindly provided by Dr A. Kispert [2] . Flag-kctd10 was generated by amplifying the zebrafish kctd10 sequence using the primer pair 5′-ATTTGCGGCCGCTATGGAAGAGATGTCAG-3′ and 5′-GAAGATCTGCGTAACTGAAGCG CTGGT-3′. The resulting PCR fragment was ligated into the NotI and BamHI sites of the p3 × FLAG-CMV-7.1 (Sigma) plasmid. The mouse Kctd10 expression vector that was used in reporter assay was constructed by amplifying the mouse Kctd10 sequence using primers 5′-CCAAGCTTTTCATGGAAGAGATGTCA-3′ and 5′-AAGATATCACTGGTGGAGGTGGG CCC-3′. The resulting PCR fragment was ligated into the HindIII and EcoRV sites of the p3 × FLAG-CMV-7.1. Human KCTD10 was amplified with primers 5′-GAAGATCTCCTG CGTCCTCCGACTTTT-3′ and 5′-AACTGCAGCTGGTGGAGGT GGGCCCG-3′ and ligated into the BglII and PstI sites of pEGFP-N1 (Clontech). To generate the Anf (−0.7)-luciferase reporter, the 0.7-kb upstream fragment of the mouse Anf gene was amplified by PCR using the primers 5′-AAGGTACCCATCCTGTTGGCACCTTG-3′ and 5′-CACTCGAGTTTGCTGTCTCTGCCCAC TC-3′, the fragment was then ligated into the XhoI and KpnI sites of pGL3 vector (Promega). HA-tbx5a was generated by amplifying the zebrafish tbx5a sequence using the primers 5′-ATTTGCGGCCGCTATGGCGGACAGTGAAG-3′ and 5′-GATCGTCGACCTGCATGTTAGC TGGC-3′; mouse Tbx5 which was used in reporter assay was amplified with 5′-ATGCGGCCG CGATACAGATGAGGGCTT-3′ and 5′-GCGTCGACAGGTCAGCCTTTAGCTATTC-3′; human: 5′-ATGCGGCCGCAGTTGGAGAGCAGAACCTT-3′ and 5′-GCGTCGACGTCTGTTGTGAAGC AGGCCTCA-3′. The resulting PCR fragments were ligated into the NotI and SalI sites of pCMV-3 × HA Hygro plasmid. Positional cloning We mapped the 34c locus to linkage group 5 using a panel of 119 microsatellite markers selected from the publicly available zebrafish genetic map [43] . For fine-mapping, 684 mutant embryos were screened with simple sequence length polymorphisms and restriction fragment length polymorphism markers. The complementary DNA of the 10 genes in the critical interval was then sequenced and analysed. Morpholino and mRNA injections Morpholino antisense oligonucleotides were dissolved in water at a concentration of 1 mM. The amount of the MOs used for injection was as follows: kctd10 MO, 4 ng per embryo; tbx5a MO, 5 ng per embryo; has2 MO, 6 ng per embryo. For each embryo, 1 nl of MO solution was injected into the cytoplasm. The sequence of MOs are: kctd10 ATG MO, 5′-TCTCTTCCATAGAAATTCCCCGATT-3′; has2 MO, 5′-AGCAGCTCTTTGGAGATGTCCCGTT-3′; tbx5 MO, 5′- GAAA GGTGTCTTCACTGTCCGCCAT-3′ (Gene Tools) [44] , [45] . Full-length capped zebrafish kctd10 mRNA was prepared using the SP6 mMessage mMachine kit (Ambion). For rescue assay, the MO against tbx5 or has2 was injected into the cytoplasm of one-cell stage embryos derived from the in-cross of Tg ( cmlc2:EGFP ) 34c+/− . The samples used for heart visualization or in situ hybridization were all genotyped for the status of kctd10 gene after observation. In situ hybridization Whole-mount in situ hybridization using digoxigenin-labelled antisense RNA probes were performed according to the standard protocols [46] . Briefly, the embryos were fixed in 4% paraformaldehyde at 4 °C overnight, and then dehydrated with alcohol. After the treatment of proteinase K, the embryos were put into the pre-hybridization buffers and incubated for 2~5 h at 65 °C. Then the probe was added into the buffer and incubated at 65 °C overnight. After washing, the samples were incubated with phosphatase-conjugated antibody against digoxigenin at 4 °C overnight. The next day, the samples were stained with NBT (Nitro Blue Tetrazolium)-BCIP (X- phosphate) (C3206, Berotime). Stained embryos were transferred into 3% methylcellulose (Sigma) and photographed under Imager A1 microscope (Zeiss) equipped with a digital camera (AxioCam MRc 5, Zeiss). The isolation of zebrafish heart and deep sequencing The hearts were isolated from the wild-type fish and the kctd10 mutant fish under the background of Tg (cmlc2:EGFP) as described previously [47] . Briefly, embryos of Tg ( cmlc2:GFP ) suspended in the ice-cold L-15 Medium (Invitrogen, Carlsbad, CA, USA) containing 10% fetal bovine serum (Hyclone, Logan, UT, USA) and Tricaine were sucked into a 1 ml needle-free syringe (Shanghai Zhiyu medical material Co Ltd). The needle was added to the syringe and the medium containing the embryos in the syringe was immediately expelled into a new dish containing the same medium. The intact GFP + hearts were identified and picked up with a p20 micropipet under fluorescent light. Total RNAs from wild-type and kctd10 mutant fish hearts were isolated with RNeasy Mini Kit (Qiagen), purified with RNeasy columns (QIAGEN). Next-generation sequencing libraries were prepared with the Illumina TruSeq preparation kit (Illumina) according to the manufacturer’s protocol and sequenced by the Illumina Hiseq 2000 platform. Around 200 million 50-bp single-end reads were obtained per sample. Reads were aligned to zebrafish genome Zv9 using tophat [48] , with up to two mismatches allowed. Differential expression analysis was performed using DESeq [49] . TALEN construction and microinjection The pair of TALENs recognizing the exon 3 of zebrafish kctd10 was designed using TALE-NT [50] and the TAL effector repeats were constructed by ‘unit assembly’ [51] . TALEN mRNA was synthesized by in vitro transcription using SP6 mMESSAGE mMACHINE Kit (Ambion). The fragments containing the TALEN target site was amplified by PCR and digested with HpaII to examine the efficiency of TALENs and to determine the phenotype in F 1 . The primers used are: Forward 5′-TGTGTGCTTCTGCAACATCCT-3′; Reverse 5′-GACACTCATCTACCAGGCCC-3′. Transfections of culture cells and reporter assays 293T cells (American Type Culture Collection, ATCC) were cultured in DMEM (Dulbecco’s modified Eagle’s medium) containing 10% fetal bovine serum (Hyclone) and 100 units ml −1 of penicillin/streptomycin (Invitrogen). Cells were plated in 24-well plates, then co-transfected with 300–500 ng of each expression vector and 100 ng of the reporter plasmid using Lipofectamine 2000 (Invitrogen). The amount of total DNA was equalized by the addition of empty expression vectors. Cells were harvested 24 h after transfection. Luciferase activity was measured using the Dual-Luciferase Reporter Assay System (Promega) according to the manufacturer’s instructions. At least three independent experiments were performed for each assay and each experiment was performed in quadruplicate. Statistical significance was determined using a Student’s t -test. Co-immunoprecipitation The whole-cell lysates of HeLa cells (ATCC) were incubated with 2 μg anti-TBX5 (bs-2354R, Bioss Inc.), 2 μg anti-KCTD10 (LS-C30750, LifeSpan Bioscience) for 12 h at 4 °C with end-over-end rotation, respectively. Protein A/G agarose beads were added and the reaction mixtures were further mixed for 3 h at 4 °C. After washed with lysis buffer for five times, proteins were extracted from the agarose beads by boiling in 2 × SDS gel-loading buffer and resolved on SDS-polyacrylamide gels. Western blotting was performed with anti-TBX5 (BIOSS) and anti-KCTD10 (LifeSpan Bioscience), respectively. 293T cells cultured in 10 cm dishes were transfected with HA-tbx5/5a and Flag-kctd10 expression constructs. After 36 h, cells were washed once with PBS and harvested. Total cell extracts were prepared in cell lysis buffer (20 mM Tris–HCl, pH 7.5, 150 mM NaCl, 10 mM NaF, 20 mM β-glycerophosphate, 1 mM sodium orthovanadate, 1 mM PMSF, 10 μg ml −1 leupeptin, 2 μg ml −1 aprotinin, 1% Triton X-100 and 1 mM EDTA). Cell lysate were mixed with HA or Flag antibodies at 4 °C for 4 h. Then lysates were incubated with Protein A and Protein G agarose (GE Healthcare) for an additional 1 h. Immune complexes were washed five times with lysis buffer. The immunocomplexes were resolved by SDS–polyacrylamide gel electrophoresis (PAGE), and western blotting was performed with the following antibodies: anti-Flag M2 (Sigma); anti-HA (Y-11) (Santa Cruz Biotechnology); anti-KCTD10 (LSBio); horseradish peroxidase-conjugated goat anti-mouse, anti-rabbit antibody (Thermo). A431 cells (ATCC) were transfected with HA-TBX5 expression construct. After 36 h, cells were washed once with PBS and harvested. Total cell extracts were prepared in cell lysis buffer (20 mM Tris–HCl (pH 7.5), 150 mM NaCl, 10 mM NaF, 20 mM β-glycerophosphate, 1 mM sodium orthovanadate, 1 mM PMSF, 10 μg ml −1 leupeptin, 2 μg ml −1 aprotinin, 1% Triton X-100 and 1 mM EDTA). Cell lysates were mixed with HA antibodies at 4 °C for 4 h. Then lysates were incubated with Protein A and Protein G agarose (GE Healthcare) for an additional 1 h. Immune complexes were washed five times with lysis buffer. Immunocomplexes were resolved by SDS–PAGE, and western blotting was performed with anti-HA antibody (Y-11) (Santa Cruz Biotechnology). GST Pull-down assays E scherichia coli BL21 harboring expression vectors for GST-kctd10 , His-tbx5a , or GST alone, His-tbx5a were grown to A 600 =0.6~0.8 and induced with isopropyl β-D-1-thiogalactopyranoside for 6 h. Purified His-Tbx5a from E. coli BL21 was incubated with GST or GST-Kctd10 bound to glutathione–Sepharose beads. The beads were collected by centrifugation and washed five times with PBS. Proteins retained on the beads were then blotted with the anti-His antibody (1:500; Santa Cruz Biotechnology). Immunofluorescence staining 293T cells grown on coverslips in six-well plates were transfected with KCTD10-EGFP and HA-TBX5 expression constructs. After 36 h, cells were washed once with PBS and fixed with 4% formaldehyde in PBS for 10 min at room temperature. Cells were then rinsed with PBS, incubated with blocking solution (0.2% Triton X-100, 3% bovine serum albumin and 1 mM NaN 3 in PBS) for 30 min at 37 °C and incubated with 2 μg ml −1 HA antibody in blocking solution for 4 h. For immunostaining of Kctd10 in zebrafish embryos, the sample was fixed with 4% formaldehyde in PBS overnight at 4 °C, then treated with blocking solution containing 0.2% Triton X-100 (v/v) for 2 h and incubated with the antibody against KCTD10 (1:300; LSBio, LS-C30750) overnight at 4 °C. After washed four times with PBS, the specimen was incubated with 20 μg ml −1 of goat anti-rabbit antibody (Alexa Fluor 594, Invitrogen) in blocking solution for 1 h, and then washed four times with PBS. The cells were incubated with DAPI (1 μg ml −1 ) in washing solution for 2 min and mounted in 90% glycerol and sealed with nail polish. Hyaluronan staining As described above, the, the hearts were isolated from the wild-type fish and the kctd10 mutant fish under the background of Tg ( cmlc2:EGFP ). The hyaluronan was stained as described [52] . Briefly, the tissue was fixed in acid-formalin-ethanol fixative (3.7% formaldehyde-PBS, 70% ethanol and 5% glacial acetic acid, all v/v) for 30 min, blocked in 1% bovine serum albumin containing 0.2% Triton X-100 (v/v) for 30 min at room temperature, then incubated with biotinylated hyaluronan-binding protein (HABP) (EMD/Millipore/Calbiochem #385911, diluted to 5 mg ml −1 ) at 4 °C overnight. After four washes with PBS, the samples were treated with Fluorescent Streptavidin Construct (Alexa Fluor 488 conjugate, Molecular Probes, S-11223, diluted to 2 μg ml −1 ) at room temperature for 2 h. The specimen was incubated with DAPI (1 μg ml −1 ) in washing solution for 20 min and washed the samples for four times. All the fluorescence samples were visualized under a fluorescence microscope (Axioimager Z1; Zeiss, Germany) or confocal laser scanning microscopes (LSM-710NLD & Duo Scan). Pharmacology and quantification of heart rate Adrenaline, digilanid and atropine were provided by Peking University Hospital. The embryos of 24 hpf derived from the incross of kctd10 +/− zebrafish were treated with adrenaline (250 μM), atropine (100 μM) and digilanid (10 μM), respectively [53] , [54] , [55] . After incubating at 28 °C for 24 h, the larvae were anesthetized with MS-222 (ethyl-3-aminobenzoate methanesulfonate salt, Sigma-Aldrich Inc.) at 28 °C. After 5 min, the images of the larvae were captured by a digital video camera attached to the microscope (Camtasia Studio) and the heart rate was calculated from the captured images [53] , [56] . Scanning Ion-selective Electrode Technique SIET [57] was used to measure extracellular K + flux at the surface of zebrafish larvae heart with a potassium-specific electrode. The assay was performed at room temperature in a small petridish filled with 1 ml PBS. The larvae hearts labelled with GFP were isolated as described above. For each sample, three different areas of the heart surface were measured. Accession codes: Deep sequencing data has been deposited in Gene Expression Omnibus under accession number GSE53022 . How to cite this article: Tong, X. et al. Kctd10 regulates heart morphogenesis by repressing the transcriptional activity of Tbx5a in zebrafish. Nat. Commun. 5:3153 doi: 10.1038/ncomms4153 (2014).